Probing failure susceptibilities of earthquake faults using small-quake tidal correlations Mitigating the devastating economic and humanitarian impact of large earthquakes requires signals for forecasting seismic events. Daily tide stresses were previously thought to be insufficient for use as such a signal. Recently, however, they have been found to correlate significantly with small earthquakes, just before large earthquakes occur. Here we present a simple earthquake model to investigate whether correlations between daily tidal stresses and small earthquakes provide information about the likelihood of impending large earthquakes. The model predicts that intervals of significant correlations between small earthquakes and ongoing low-amplitude periodic stresses indicate increased fault susceptibility to large earthquake generation. The results agree with the recent observations of large earthquakes preceded by time periods of significant correlations between smaller events and daily tide stresses. We anticipate that incorporating experimentally determined parameters and fault-specific details into the model may provide new tools for extracting improved probabilities of impending large earthquakes. The viability of using tidal correlations as a predictive measure for earthquakes has been controversial, as only 1% of the earthquakes seem to correlate significantly with tides [1] , [2] . It is estimated that tens or hundreds of thousands of earthquakes must be analysed to detect significant correlations with tides [2] , [3] . Focusing on correlations between large earthquakes and tidal stresses is thus not likely to be practical. On the other hand, small earthquakes are much more numerous than large ones. Therefore, detecting significant correlations between small earthquakes and periodic stresses may be feasible on timescales relevant to hazard prevention. Small quakes are expected to increase in number as the stress on a fault increases [4] , [5] . However, observed small earthquake rates fluctuate strongly in time because of episodic occurrence of aftershocks of moderate and small local events, triggered seismicity from large remote earthquakes and other transients. This has precluded forecasting the onset of large earthquakes using predictive measures based on number of events alone [6] , [7] , [8] , [9] . On the other hand, predictive measures that are less sensitive to transient effects and track the evolving response of a fault to repeating forcing terms could prove useful. For instance, ongoing oscillatory loadings like tidal stresses may be viewed as ‘repeating’ probes that can be used to test the evolving susceptibility of a given fault system. Transient effects uncorrelated with the stress oscillations will cancel out in analyses based on correlations. Several recent studies have detected significant correlations between the occurrence of small seismic or volcanic events and periodic stresses, such as daily tide stresses [10] , [11] , [12] , [13] , [14] and seasonal loadings [15] , [16] . Tanaka [12] , [13] analysed observational earthquake data before large earthquakes observed in Indonesia and Japan, and found that correlations between small seismic events and daily tide stresses increased just before these large events. These precursory correlations could be indicative of the fault being pushed past a critical state into a regime of higher susceptibility [17] , [18] . However, there is limited experimental evidence that increases in correlations of tidal or seasonal triggering with small earthquakes tend to occur before large earthquakes. This is, in part, because laboratory experiments on sheared rocks have mostly focused on correlations of oscillatory stresses with large stick-slip events (analogous to large earthquakes [2] , [3] , [19] . To build physical intuition about the basic mechanisms of earthquake triggering, we construct a simple probabilistic model from a framework that accounts for various features of earthquakes and plasticity [6] , [20] , [21] , [22] , [23] , [24] . We use the model to compute probabilities of large earthquakes from correlations between the timings of small earthquakes and periodic fault stresses, such as tidal or seasonally varying loadings [1] , [10] , [11] , [15] , [16] . The goals of this study are to use the model to determine the essential features of earthquake faults and small earthquake statistics that lead to correlation patterns like those observed by Tanaka; to estimate the probability of impending large earthquakes from the measured correlations; and finally, to motivate future analyses of correlations between periodic stresses and small earthquakes on natural faults and in laboratory experiments. Despite the simplicity of the model, we find good agreement with the observed trends of correlations of natural earthquakes with tidal stresses, and make predictions on additional refined features that may be tested with future data. The model Our model qualitatively reproduces the correlation behaviours observed by Tanaka, suggesting that correlations between small earthquakes and daily tide stresses can in principle be used to gauge whether the fault is in a critical state (that is, can generate a large event) and estimate the probability of impending large earthquakes. We briefly describe the model here. 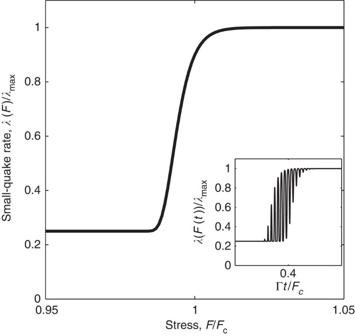Figure 1: Small earthquake rate as a function of stress and time. For stresses much less than the critical stress of the fault,Fc, the rateλ(F) of small earthquake occurrences is low, rising quickly as the stress approachesFcbefore leveling off at higher stresses. The stress-dependent probability that a small event triggers a large event has a qualitatively similar shape. Inset: if the fault is subjected to periodically varying stresses in addition to regular slow tectonic shear, the small event rate will exhibit oscillations in time. An oscillation frequency much smaller than real daily tide stress frequencies has been used so that oscillations may be clearly seen in the plot. Figure 1: Small earthquake rate as a function of stress and time. For stresses much less than the critical stress of the fault, F c , the rate λ ( F ) of small earthquake occurrences is low, rising quickly as the stress approaches F c before leveling off at higher stresses. The stress-dependent probability that a small event triggers a large event has a qualitatively similar shape. Inset: if the fault is subjected to periodically varying stresses in addition to regular slow tectonic shear, the small event rate will exhibit oscillations in time. An oscillation frequency much smaller than real daily tide stress frequencies has been used so that oscillations may be clearly seen in the plot. 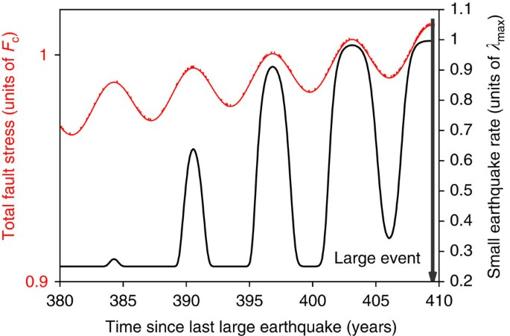Figure 2: Stress versus time on a simulated fault, along with the small event rate. The total average stressF(t) on the fault (red curve) increases linearly in time and is perturbed by an oscillatory stress. The small vertical dashes on the curve represent times at which small earthquakes occurred. Note the accumulation of events near peaks in the stress. The black curve represents the variation of the small event rateλ(F(t)) as the stress varies on this fault. When the total stress approaches a critical valueFc, a large earthquake occurs, releasing the built-up stress to the surroundings. The fault stress quickly relaxes to a baseline stress levelf(equal to 0.595Fcin this figure), before accumulating stress again. The small event rate is similarly reduced to the minimum rate. An oscillation frequency much lower than real daily tide stress frequencies has been used so that oscillations may be clearly seen in the plot. Full size image Figure 2: Stress versus time on a simulated fault, along with the small event rate. The total average stress F ( t ) on the fault (red curve) increases linearly in time and is perturbed by an oscillatory stress. The small vertical dashes on the curve represent times at which small earthquakes occurred. Note the accumulation of events near peaks in the stress. The black curve represents the variation of the small event rate λ ( F ( t )) as the stress varies on this fault. When the total stress approaches a critical value F c , a large earthquake occurs, releasing the built-up stress to the surroundings. The fault stress quickly relaxes to a baseline stress level f (equal to 0.595 F c in this figure), before accumulating stress again. The small event rate is similarly reduced to the minimum rate. An oscillation frequency much lower than real daily tide stress frequencies has been used so that oscillations may be clearly seen in the plot. Full size image The basic model assumptions are: 1 The earthquake fault slips in two classes of seismic events: (a) ‘small to moderate earthquakes’, which have sizes distributed according to Gutenberg–Richter statistics, up to some maximum (‘cutoff’) size and (b) large ‘characteristic earthquakes’, which have sizes narrowly distributed about some large magnitude that exceeds the cutoff size of the small earthquakes. The exact values of the cutoff magnitude of the small-moderate earthquakes and the magnitude of the large earthquakes depend on fault details, such as geometrical parameters and degree of heterogeneity [4] , [18] ; for example, on the San Andreas Fault, large characteristic earthquakes have magnitudes of ~7.5 or more [25] , [26] . 2 Small earthquakes occur randomly at an average rate λ ( F ), which depends on the (average) fault shear stress, F = F ( t ), where t is the time since the previous large earthquake. We assume that λ ( F ) is small for fault stresses F much less than a critical stress level, F c , and rises rapidly to a larger rate as F → F c . This behaviour is shown in Fig. 1 . Figure 2 demonstrates how the stress F ( t ) and the rate λ ( F ( t )) of small earthquakes vary together with time. 3 A small earthquake can trigger a large earthquake according to a stress-dependent probability, P ( F ). The function P ( F ) is small for stresses less than the critical stress F c , and rises sharply to 1 as the total fault stress approaches F c (see Supplementary Methods for details). 4 Stress drops due to large earthquakes cause the average fault stress, F ( t ), to relax to a baseline value, f , immediately after a large quake, as seen in Fig. 2 (ref. 18 ). In contrast, stress drops caused by small earthquakes can be neglected in analyses focusing on large scales. This is because they affect only small areas of the fault, and therefore, to first approximation, do not significantly change the fault-averaged stress F ( t ). (Note: in this paper, we measure stresses in units of a ‘typical stress drop’, F c − f , rather than the critical stress F c , since F c is difficult to measure in real faults. As parameters for the simulations, we use estimates of the relative strengths of F c and f from laboratory experiments designed to mimic earthquake faults). Origins of the model assumptions Our assumptions are probabilistic formulations of the physical assumptions of a simple microscopic model of earthquake dynamics and plasticity [6] , [20] , [21] , [22] , [23] , [24] . In this microscopic model, weak spots along a fault slip under slow shear, which redistributes stress to nearby weak spots, and may cause them to slip as well, resulting in a slip-avalanche, or earthquake. In addition, the model incorporates a dynamic weakening effect where the threshold stress for a spot to slip is reduced after its initial slip in a given failure episode, and returns to normal once the earthquake is arrested. The microscopic model produces a wide range of event sizes, which in the probabilistic model are grouped into ‘small-moderate’ and ‘large’ event sizes. The large earthquakes on a relatively homogenous fault occur almost periodically in time, are of a characteristic magnitude and span the entire fault. The small-moderate events occur in between the large events, are irregularly spaced in time and have power law distributed magnitudes [4] , [6] , [18] . The assumption that the rate of small event activity increases with increasing stress emerges naturally from this simple model and has been observed in earthquake faults [5] , deformation experiments [27] , [28] and other models [4] , [20] , [21] , [22] , [23] , [24] . (As mentioned above, however, transient effects from the surrounding region or other fault sections obscure the observed increase of event rates, rendering observed rates alone insufficient to predict the onset of impeding large earthquakes [7] , [8] ). The other three assumptions also result from the microscopic model [6] , [20] , [21] , [22] , [23] , [24] . The underlying microscopic model predicts the universal (that is, detail-independent) statistical features of many sheared stick-slip systems, including earthquake size distributions [4] , [20] , [21] , [22] , [29] and size distributions of slip-avalanches in sheared nanosized crystals [27] , amorphous materials [28] and granular matter [23] , [24] . The microscopic model and its probabilistic formulation capture the basic features, rather than the fine details of each earthquake fault and hence may only yield qualitative predictions of some statistical observations. However, our model is expected to fully predict the universal aspects of the statistics and to provide an understanding of the fundamental physics behind tidal or seasonal earthquake triggering. More detailed models building on the simple model (for example, see the model of ref. 15 ) can be used to also address fault-specific questions, but at the price of adding more parameters that are not well constrained. In the presence of tidal or seasonal stresses acting on the fault, the stress F ( t ) has two main contributions: an ongoing loading stress that increases at a slow constant rate Γ caused by the slow motion of tectonic plates and an additional perturbative periodic stress resulting from the tidal or seasonal stresses ( Fig. 2 ). Our first goal is to detect correlations between the small earthquakes and the periodic component of F ( t ), and verify that the model can produce increased correlations before large earthquakes, as seen in real fault data by Tanaka [12] , [13] . Correlation analysis As the stress on the fault evolves in time, the model generates a time series of small earthquakes interrupted by recurring large earthquakes. We analyze this time series for correlations using similar methods as Tanaka [12] , [13] . We use daily tidal stresses of a single amplitude in our analyses; we thus refer to the daily tidal stresses as diurnal rather than semidiurnal, though we expect similar results for both. Annual tidal amplitudes are an order of magnitude smaller, so we do not consider them here. See the Methods section, Supplementary Methods and Supplementary Table 1 for details. We identify correlations between small earthquakes and diurnal tide stresses by recording the phase of the periodic stress at which each earthquake occurs. If most earthquakes occur near a preferred phase, the correlations are strong. Following Tanaka, we use a P value test statistic as a quantitative measure of correlation. Suppose we measure a non-uniform histogram of phases at which the small earthquakes occur. The P value is then the probability that we observe at least as non-uniform a histogram of phases, given that the small earthquakes are triggered completely randomly. When the P value <5–10%, there is a low probability that completely random triggering would generate the observed phase histogram; hence, the correlations are strong. When the P value >10%, the correlations are weak or non-existent. The P value varies with time and depends on the number of earthquakes recorded per unit time. As the fault stress nears the critical stress, the rate λ ( F ) of small earthquake occurrences begins to track the stress F ( t ) ( Figs 1 and 2 ), and the P value tends to drop, indicating the fault’s increased susceptibility to external stress changes, resulting in stronger correlations. To evaluate the effectiveness of the P value as a predictor of large earthquakes, we perform two analyses. First, we determine the range of periodic stress amplitudes for which strong correlations (small P values) are observed in the model. We do so by comparing the distribution of P values when a large earthquake occurs, for stress amplitudes up to 10% of the estimated typical stress drop, F c − f . We find amplitudes around 1.2–2.5% of the stress drop are the smallest that result in significant correlations ( P values <10%) between the periodic driving and earthquake triggering, so we focus on these amplitudes in our next analysis: we smooth the P value curve and compute the probability that a large earthquake occurs within a specified amount of time after the smoothed P value dips below a desired threshold value. A set of four runs of the simulated P value versus time between two large earthquakes for which significant correlations are observed is presented in the first column of Fig. 3 . The second column of Fig. 3 displays the phase distribution of the last 100 small events in each run before the large earthquake occurs. The third and fourth columns of Fig. 3 present the P value and phase histogram data, respectively, adapted from Tanaka [12] , [13] . Qualitatively, the behaviour of the simulations agrees well with the observed P values. 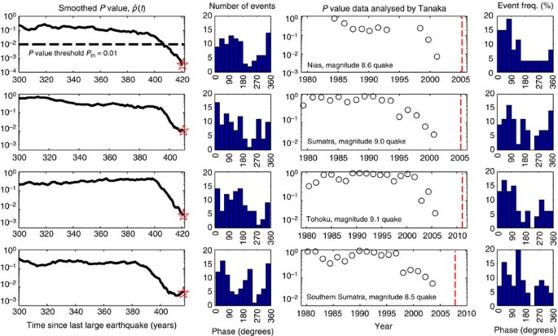Figure 3: Simulated and observedPvalue curves and phase histograms for small quakes. First column: four examples in which the smoothedPvalue,, in our simulations indicates significant daily tide correlations as it varies between large earthquakes, for a (diurnal) tidal stress amplitude of 2.5% of the stress drop. Second column: the simulated distribution of phases of the last 100 small earthquakes that occurred before the large earthquake was triggered. The red stars in the first column indicate when the large earthquake occurred. In the first plot of the first column, an example threshold ofPth=0.01 is shown (dashed black line). Third and fourth columns:Pvalue variation and phase histograms of the small earthquakes that occurred 3,000 days before the large earthquakes, as seen in observational data from three faults in Indonesia (Sumatra, Southern Sumatra and Nias) and a fault in Japan, adapted from refs12,13. The dashed red lines in the third column plots indicate when the large earthquake occurred on those faults. The qualitative agreement between the simulations is excellent for a minimal model that only captures the essential details of earthquake statistics on a fault. Small values of thePvalue indicate strong correlations between small earthquakes and the periodic component of the fault stress. As the large earthquake is approached, thePvalue drops significantly, indicating strong correlations between the timing of small earthquakes and tidal stresses. Labels of theyaxes are given as the titles in each column. Figure 3: Simulated and observed P value curves and phase histograms for small quakes. First column: four examples in which the smoothed P value, , in our simulations indicates significant daily tide correlations as it varies between large earthquakes, for a (diurnal) tidal stress amplitude of 2.5% of the stress drop. Second column: the simulated distribution of phases of the last 100 small earthquakes that occurred before the large earthquake was triggered. The red stars in the first column indicate when the large earthquake occurred. In the first plot of the first column, an example threshold of P th =0.01 is shown (dashed black line). Third and fourth columns: P value variation and phase histograms of the small earthquakes that occurred 3,000 days before the large earthquakes, as seen in observational data from three faults in Indonesia (Sumatra, Southern Sumatra and Nias) and a fault in Japan, adapted from refs 12 , 13 . The dashed red lines in the third column plots indicate when the large earthquake occurred on those faults. The qualitative agreement between the simulations is excellent for a minimal model that only captures the essential details of earthquake statistics on a fault. Small values of the P value indicate strong correlations between small earthquakes and the periodic component of the fault stress. As the large earthquake is approached, the P value drops significantly, indicating strong correlations between the timing of small earthquakes and tidal stresses. Labels of the y axes are given as the titles in each column. Full size image There are some quantitative differences between our simulations and real data. For example, the timescale over which the P value drops, and hence the relevant timescales for hazard preparedness, is about 20 years in our simulations, compared with 5–10 years in Tanaka’s observations. In our model, this timescale is primarily set by the ratio Γ/( F c − f ), the slow loading rate Γ over the average stress drop ( F c − f ) resulting from a large earthquake, and the range of stresses over which the small event rate increases. In natural faults, features not captured by our model, such as fault geometry and some aseismic slip, may also influence this timescale. Our model also produces slightly more significant correlations (lower P values) than those presently observed in real data. This could be due to a number of factors, including the higher complexity of natural faults and differences in the details of the small event rate on natural faults. Nonetheless, the qualitative agreement between our simulations and the observational data demonstrates that our model captures the essential statistical physics of the earthquake faults. For modelled diurnal tide variations with amplitudes <1% of F c − f , the P values obtained just before large earthquakes occur are statistically similar to the P values obtained in the absence of any periodic stressing, indicating weak correlations ( Fig. 4 ; see also Supplementary Figs 1 and 2 ). For faults subject to such small oscillatory stresses, additional analyses (using, for example, Bayesian inference) may boost the signal to make the P value a more reliable earthquake probability predictor. However, for faults subject to slightly larger oscillatory stresses (>1.2–2% of the stress drop), the correlations are readily apparent, and the P value could be a useful predictor of large quakes. The faults in Tanaka’s observations of tidal triggering experienced oscillatory stresses of ~10 3 –10 4 Pa (ref. 12 ); for typical stress drops on the order of MPa, these amplitudes are about 0.1–1% of the typical stress drop on a fault. This is slightly smaller than our model predicts. However, we considered only oscillations in shear stress. In nature, oscillatory loadings produce changes in both shear and normal stresses. At locations where the shear stress increases and the normal stress decreases, the effect will be amplified. In addition, stress drops fluctuate by several orders of magnitude (see, for example, ref. 30 ), so even ~2.5% of the mean stress drop may overestimate the amplitude needed to trigger a large earthquake in some faults. Local fault conditions not captured by our model, such as depth of the earthquake source and details of the small earthquake rate, may also influence the actual stress amplitudes needed to trigger large earthquakes. While the same effects may, in some cases, increase the necessary tidal amplitude for triggering large earthquakes, our results demonstrate that it is possible for oscillatory stresses of modest amplitudes to trigger large earthquakes in some circumstances. Furthermore, we found that the correlations between small earthquakes and tidal stresses provide a potential proxy for the susceptibility of the fault to failure. Most experimental work to date has focused on finding correlations between large earthquakes and tides. Our results provide motivation for looking more closely at correlations between tidal stresses and small earthquake occurrences in laboratory experiments and natural settings. We have focused on results for diurnal tide stresses here, but we expect similar results for seasonal-stress variations; see the Supplementary Discussion , Supplementary Table 1 and Supplementary Fig. 3 for preliminary results. 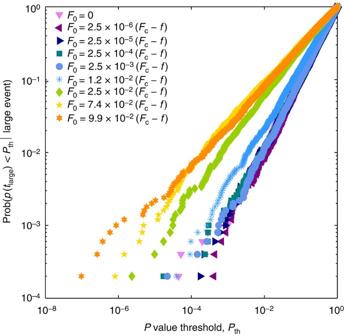Figure 4: Cumulative probability distribution ofPvalues when large earthquakes occur. The vertical axis of this plot represents the cumulative distribution ofPvalues observed when the large earthquake occurs in our simulations. In the absence of diurnal tide stresses (F0=0), and for diurnal tide stresses with amplitudes less than 1% of the typical stress drop caused by a large earthquake,Fc−f, thePvalue is >0.1 over 90% of the time when a large earthquake occurs, and most data points for these amplitudes lie approximately along the same line. For these amplitudes, thePvalue is not a statistically significant predictor of large earthquakes. However, for amplitudes≳1.2–2.5% of the stress drop, there is a significant probability that thePvalue will be below 0.1 when the large earthquake occurs, indicating significant correlations between the earthquakes and tides. For faults subject to strong tidal or seasonal amplitudes relative to the stress dropFc−f, thePvalue may thus be useful for estimating the risk of large earthquakes. The amplitudes given in the legend have been converted from units of critical stressFcto units of typical stress dropFc−f, using the relationFc−f=0.405Fc(seeSupplementary Methodsfor parameter values). In the original units of critical stress, the amplitudes are 0, 10−6, 10−5, 10−4, 10−3, 5 × 10−3, 10−2, 3 × 10−2and 4 × 10−2Fc. Figure 4: Cumulative probability distribution of P values when large earthquakes occur. The vertical axis of this plot represents the cumulative distribution of P values observed when the large earthquake occurs in our simulations. In the absence of diurnal tide stresses ( F 0 =0), and for diurnal tide stresses with amplitudes less than 1% of the typical stress drop caused by a large earthquake, F c − f , the P value is >0.1 over 90% of the time when a large earthquake occurs, and most data points for these amplitudes lie approximately along the same line. For these amplitudes, the P value is not a statistically significant predictor of large earthquakes. However, for amplitudes ≳ 1.2–2.5% of the stress drop, there is a significant probability that the P value will be below 0.1 when the large earthquake occurs, indicating significant correlations between the earthquakes and tides. For faults subject to strong tidal or seasonal amplitudes relative to the stress drop F c − f , the P value may thus be useful for estimating the risk of large earthquakes. The amplitudes given in the legend have been converted from units of critical stress F c to units of typical stress drop F c − f , using the relation F c − f =0.405 F c (see Supplementary Methods for parameter values). In the original units of critical stress, the amplitudes are 0, 10 −6 , 10 −5 , 10 −4 , 10 −3 , 5 × 10 −3 , 10 −2 , 3 × 10 −2 and 4 × 10 −2 F c . Full size image We find that when our model fault is subjected to a diurnal tide stress with sufficiently large but still modest amplitudes (greater than 1% of the stress drop in the model), the behaviour of the (smoothed) P value can be used to predict how likely future earthquakes are. 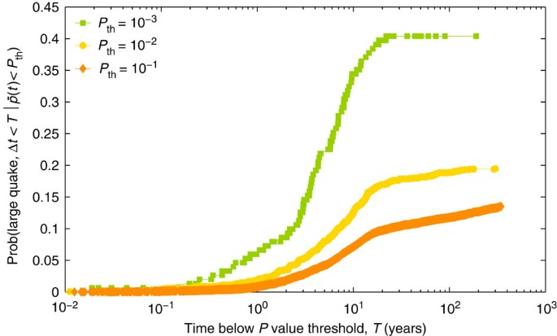Figure 5: Simulated probabilities that a large earthquake will occur. Here we plot the probability that a large earthquake occurs within a time Δt<Tafter the smoothedPvalue curve,, descends below a threshold levelPth. The (diurnal) tidal amplitude used is 2.5% of the stress drop. Each curve corresponds to a differentPththreshold. For example, ifis observed to descend belowPth=10−3(green squares), there is a 34% chance that a large earthquake will occur within 10 years, assumingdoes not rise above the threshold level before the large quake occurs. The curves become more sparsely sampled at lower thresholds, asdips below the smaller thresholds less often, so we show only the best estimated probabilities. We also compute the distribution of waiting times from the first observation that thePvalue descends below the thresholdPthto the time the large earthquake occurs; see theSupplementary Discussionfor details. Figure 5 displays the simulated probability that a large earthquake occurs within a time T after the P value dips below a threshold value P th . For example, if we observe that the P value dips below P th =10 −3 (green squares), a large earthquake has a 34% chance of occurring within 10 years, assuming the P value does not increase above 10 −3 before then. See Supplementary Fig. 4 for results of an analysis of the probability of a large earthquake occurring within T years after observing the P value dip below the threshold P th at least once. Figure 5: Simulated probabilities that a large earthquake will occur. Here we plot the probability that a large earthquake occurs within a time Δ t < T after the smoothed P value curve, , descends below a threshold level P th . The (diurnal) tidal amplitude used is 2.5% of the stress drop. Each curve corresponds to a different P th threshold. For example, if is observed to descend below P th =10 −3 (green squares), there is a 34% chance that a large earthquake will occur within 10 years, assuming does not rise above the threshold level before the large quake occurs. The curves become more sparsely sampled at lower thresholds, as dips below the smaller thresholds less often, so we show only the best estimated probabilities. We also compute the distribution of waiting times from the first observation that the P value descends below the threshold P th to the time the large earthquake occurs; see the Supplementary Discussion for details. Full size image This analysis method should be applicable to observed earthquake catalogues and allow, by tracking correlations with tides and observing the statistical behaviour of the P value, estimates of the risk of an impending large earthquake. The P value analysis could be complemented with other signals to develop stronger predictive techniques. For example, while previous studies using b value fluctuations and increases in the number of events before large earthquakes as predictors on their own have not yielded satisfactory results [4] , [6] , [7] , [8] , [31] , Bayesian inference analyses which combine those results with phase-distribution information studied in this work may enable boosted estimates of large earthquake risk probabilities. Our model can be adapted to include more detailed loading conditions that could affect correlation measurements, including the effects of seismic waves from nearby faults, or spatial variations of stresses along the fault, which could in turn cause spatial variations in correlations. Tanaka’s [13] study of the 2011 Tohoku earthquake indicates that correlations are only significant near the epicentre of an earthquake. Incorporating spatial information into the P value analyses may enable predictions of the most likely locations of impending large earthquake epicentres. For realistic fault conditions and laboratory experiment set-ups [2] , [3] , [4] , [19] , [32] , [33] , our model can serve as a simple testing-ground for developing new analyses or tools to be applied to data. Controlled laboratory experiments can also allow for detailed quantitative comparisons between our model predictions and observations. To achieve quantitative agreement, the experiments must be able to detect small earthquake-like slip events. The necessary quantities to measure are the observed rate ( λ ( F )) of events as the external stress or force on the system increases and histograms of the stresses at which the large slip events occur, to estimate P ( F ) (as the normalized histogram multiplied with the stress-bin size). After a quantitative characterization of these functions and other model parameters is obtained, a tailored version of our model could be simulated for the same parameters, enabling quantitative comparison between model predictions and experimental results. Combining laboratory experiments and observational data with understanding gleaned from simple models such as the one presented here may improve our ability to make quantitative estimates of the risk of large earthquakes on natural faults. Simulation of earthquake time series We simulated a time series of small earthquakes, generated by a non-homogeneous Poisson process (this is the mathematical formulation of model assumption (2)). The rate of small earthquake occurrences depends on the total stress on the fault, which varies in time due to both a slow tectonic linear shear and the external oscillatory stress of frequency ω . The exact form we chose is F ( t′ )= f +Γ( t′ − T last )+ F 0 (sin( ωt′ + ϕ 0 )−sin( ωT last + ϕ 0 )), where t′ is the absolute time from the start of the simulation, related to the time t since the last earthquake by t′ = t + T last , and T last is the time of the previous large earthquake. F ( T last )= f is the constant arrest stress after a large quake, Γ is the slow tectonic shear rate of the fault and F 0 and ϕ 0 are the amplitude and initial phase of the periodic component of the stress, respectively. As the oscillatory component has a single amplitude, it approximates a diurnal tide stress, though semidiurnal tide stresses could be straightforwardly implemented. When a small earthquake occurs, it may trigger a large earthquake with probability P ( F ). After a small earthquake successfully triggers a large earthquake, we reset the average fault stress F ( t′ ) to the constant arrest stress level f and repeat the process. For each small earthquake, we recorded the effective phase at which the earthquake occurs, ( ωt′ quake + ϕ 0 ) mod 2π , where t′ quake is the time at which the earthquake occurred and ϕ 0 is again the relative phase of the oscillatory stress at t′ =0. Analysis of earthquake time series To test the susceptibility of the fault to failure, we analysed correlations between the occurrence of small earthquakes and the oscillatory component of the external stress on the fault. We focused on oscillatory stress correlations for several reasons. As stated in the main text, oscillatory stresses may be viewed as repeating probes of the state of the fault, allowing us to test the susceptibility of the fault to failure. Predictive measures based only on the observed number of events have not proved reliable, due to transient effects such as remote seismic waves from other faults that would obscure the true rate of small earthquakes occurring on a single fault. Such remote events would not correlate with the tides, however, and would cancel out of the correlation analysis we perform here. Furthermore, any analysis of the significance of fluctuations in event rate must assume, a priori, a model for the expected number of events [14] . In contrast, the phase-correlation method that we employed only requires the natural assumption that events uncorrelated with oscillatory stressing will yield a uniform distribution of phases at which the events occur, independent of the model or process that generated those events. Thus, another reason to prefer the phase-correlation method is to keep the data analysis and model as independent as possible. To evaluate the significance of correlations between the oscillatory stresses and small earthquake occurrences, we recorded the phases of small earthquakes between two consecutive large earthquakes, and computed a corresponding P value statistic. The P value statistic we use quantifies the probability that a sequence of small earthquakes would occur with a histogram of phases at least as non-uniform as that of the observed sequence. This corresponds to the null hypothesis that small earthquakes are triggered independently of the oscillatory stress and hence the expected histogram for large numbers of phases would be uniform. Following Tanaka [12] , [13] and others [3] , [19] , [34] , we used a Schuster test to compute the P value, p ( t )=exp(− D ( t ) 2 / n ( t )), where n ( t ) is the number of events recorded at a time t since the previous large earthquake, and . Here the ϕ k are the phases of the oscillatory stress at which the small earthquakes occurred. This equation for the P value is valid only for large numbers of earthquakes, so we fixed p ( t )=1 until 200 small earthquakes had been accumulated. We reset the P value to 1 following a large earthquake. See Supplementary Fig. 5 for plots of n ( t ) and the small event rate sampled at times at which the events occur, for the cases shown in Fig. 3 . We computed the P value between 5,000 simulated large earthquakes. To test the effectiveness of both diurnal tidal correlations and seasonal-stress correlations of different amplitudes, we first recorded the values of p ( t ) at the time that the large earthquakes occur. We computed the cumulative distribution ( Fig. 4 ) of these values for several different oscillatory amplitudes ranging from 0 to 10% of the typical stress drop (or 0–4% of the critical stress F c ). We chose this amplitude range based on estimates of typical local average stress drops on faults, compared with typical tidal or seasonal amplitudes [35] , [36] . We performed this analysis for two specific frequencies: one corresponding to a diurnal tidal stress frequency of 2 π /(25 h) ( Fig. 4 ), and one corresponding to the frequency of annually varying load stresses, 2 π /(1 year) (see Supplementary Discussion and Supplementary Fig. 3 for preliminary results on the effect of yearly stress frequencies). Because actual tidal periods are longer than 24 h, we rounded up to a 25-h period. This slight difference does not affect our results in any qualitative way. Semidiurnal tidal stresses have two high and low tides, whereas diurnal tidal stresses have (approximately) a single amplitude. We used diurnal tidal stresses for simplicity, but we expect similar results for semidiurnal tidal stresses. From the above analysis, we found that amplitudes on the order of 1% or greater of the typical large stress drop on the fault correlated significantly with daily tides. We then chose one of the smallest amplitudes in this range, F 0 /( F c − f )=2.5%, to investigate the time-dependent behaviour of the P value curve between two large earthquakes, rather than just the P value at the time when the large earthquake occurred. The raw P value curve, p ( t ), exhibits many fast, small jumps; so to compute the data in Fig. 5 , we first smoothed the curve using a window of 500 days to obtain the trend line. The routine we used to smooth our non-uniformly spaced data was written by Andreas Eckner (www.eckner.com). The routine uses a constant-value interpolation between data points and integrates over the curve to perform the smoothing. We then analysed how often a large earthquake occurred when the smoothed P value, , dipped below some specified threshold P th . We recorded the length of the continuous duration, Δ t , for which was less than P th before the large earthquake occurred, or before rose above P th again. We used this data to compute the probability , shown in Fig. 5 . We also computed the probability of observing a large event within some time T after observing the smoothed P value dip below the threshold P th at least once (see Supplementary Methods ). A detailed discussion of the simulation, including functional forms of λ ( F ) and P ( F ), as well as the specific parameter values used for the various stress and timescales, is included in the Supplementary Methods . How to cite this article : Brinkman, B. A. W. et al . Probing failure susceptibilities of earthquake faults using small-quake tidal correlations. Nat. Commun. 6:6157 doi: 10.1038/ncomms7157 (2015).